High susceptibility to fatty liver disease in two-pore channel 2-deficient mice Endolysosomal organelles play a key role in trafficking, breakdown and receptor-mediated recycling of different macromolecules such as low-density lipoprotein (LDL)-cholesterol, epithelial growth factor (EGF) or transferrin. Here we examine the role of two-pore channel (TPC) 2, an endolysosomal cation channel, in these processes. Embryonic mouse fibroblasts and hepatocytes lacking TPC2 display a profound impairment of LDL-cholesterol and EGF/EGF-receptor trafficking. Mechanistically, both defects can be attributed to a dysfunction of the endolysosomal degradation pathway most likely on the level of late endosome to lysosome fusion. Importantly, endolysosomal acidification or lysosomal enzyme function are normal in TPC2-deficient cells. TPC2-deficient mice are highly susceptible to hepatic cholesterol overload and liver damage consistent with non-alcoholic fatty liver hepatitis. These findings indicate reduced metabolic reserve of hepatic cholesterol handling. Our results suggest that TPC2 plays a crucial role in trafficking in the endolysosomal degradation pathway and, thus, is potentially involved in the homoeostatic control of many macromolecules and cell metabolites. Endo/lysosomal vesicle trafficking is important for many cells and organ systems. In the liver, receptor-mediated uptake of low-density lipoproteins (LDLs) and subsequent intracellular transport is essential for hepatic cholesterol homoeostasis and plasma lipoprotein metabolism. Dysfunction within this pathway results in liver disease such as non-alcoholic fatty liver disease (NAFLD), which is associated with increased cardiovascular and liver-related mortality [1] . NAFLD is the most common cause of chronic liver disease in Western Europe and the United States [2] , [3] . It has been estimated that as many as 30% of adults in these countries have NAFLD [2] . This liver disease has thus emerged as a substantial public health concern. The spectrum of NAFLD ranges from simple lipid accumulation in hepatocytes (steatosis) in absence of alcohol, which is considered relatively benign, to steatosis with liver damage, inflammation and fibrosis (non-alcoholic steatohepatitis (NASH)) and progressive liver disease, including cirrhosis and hepatocellular carcinoma [4] . The hallmark of NAFLD is hepatic neutral lipid accumulation, mainly triacylglycerol and cholesterol ester (CE). The roles of both triglycerides and free fatty acid accumulation in NAFLD have been elucidated in many studies [5] . By contrast, the role of cholesterol in NAFLD has been less extensively studied but is gaining increasing attention [1] , [6] , [7] , [8] . Recent studies have demonstrated that cholesterol metabolism and trafficking might play an important role in the pathogenesis of NAFLD and NASH [1] . Cholesterol is highly enriched in LDLs and is taken up by the liver via receptor-mediated endocytosis of the LDL–LDL receptor complex at the plasma membrane. After internalization, membrane vesicles containing this complex fuse to early endosomes. Subsequently, LDL receptors and its ligand LDL are separated in the sorting endosome and distributed by two major routes: the recycling pathway transports LDL receptor proteins back to the plasma membrane; the degradation pathway traffics LDL to late endosomes and lysosomes. This pathway involves maturation of early endosomes into multivesicular bodies/late endosomes which finally fuse with lysosomes [9] , [10] , [11] , [12] , [13] , [14] , [15] . LDL-cholesterol exits from late endosomes and lysosomes and is either metabolized to bile acids (BAs) and excreted, stored as CEs in lipid droplets or exported from hepatocytes into the plasma. While the principle pathways of LDL transport in the endolysosomal vesicle system are well characterized, the distinct proteins involved in these processes are largely unknown. Interesting candidate proteins, which might regulate endolysosomal trafficking, and fusion processes are cation channels present in the membrane of endolysosomal vesicles. Recently identified cation channels that may generate Ca 2+ signals during endolysosomal fusion events and thereby vesicle trafficking are the two-pore channels (TPCs) [16] , [17] . Two different TPC subtypes exist in mouse and man, TPC1 and TPC2. There is evidence that TPC1 is mainly present in the proximal endosomal system, and TPC2 is predominantly expressed on late endosomes and lysosomes [16] , [18] , [19] . The activation mechanism of TPCs is complex and has been suggested to involve the second messenger nicotinic acid adenine dinucleotide phosphate (NAADP) and the endolysosomal membrane lipidphosphatidylinositol (3,5)-bisphosphate (PI(3,5)P 2 ) [17] , [18] , [20] , [21] , [22] , [23] , [24] . Independent of what the nature of the endogenous ligand of these channels might be, there is substantial evidence that on activation TPCs mediate the release of Ca 2+ from lysosomal stores. Patch-clamp [21] , [22] , [24] , lipid bilayer and calcium imaging experiments [18] , [25] , [26] indicate that TPCs are Ca 2+ permeable channels and, hence, may directly confer Ca 2+ release from endosomes/lysosomes. Here, we demonstrate that TPC2-deficient cells display profound trafficking defects in the endolysosomal degradation pathway. We provide evidence that TPC2 cation channels may directly be involved in Ca 2+ signalling necessary for endolysosomal fusion processes. On the whole-animal level, we demonstrate that loss of TPC2 leads, as a result of the observed trafficking defects, to enhanced hepatic cholesterol accumulation, hyperlipoproteinaemia, and to NASH. These findings indicate a reduced metabolic reserve of hepatic cholesterol handling. Our results suggest that TPC2 plays a crucial role in endolysosomal trafficking in the endolysosmal degradation pathway and, thus, is potentially involved in the homoeostatic control of many macromolecules and cell metabolites. Loss of TPC2 impairs trafficking in the degradation pathway To test whether TPC2 is implicated in endolysosomal trafficking, we disrupted the Tpc2 gene in the mouse ( Fig. 1a ). In this mouse line, exon 7 of TPC2, which encodes TMD5 and part of the pore-loop of domain I, is globally deleted ( Fig. 1a ). This targeting strategy results in non-functional ion-channel proteins and is different from the strategies used for two mouse lines published before [17] , [18] . The deletion of the TPC2 gene was confirmed by genomic DNA analysis using Southern blot (not shown), PCR strategies, immunocytochemistry and western blotting ( Supplementary Fig. 1a,b ). Reverse-transcription PCR (RT–PCR) revealed the absence of exon 7 of TPC2 in TPC2−/− murine embryonic fibroblasts (MEFs) and hepatocytes ( Supplementary Fig. 1b ). In addition, we generated a TPC2 antibody to detect TPC2 protein. In agreement with the RT–PCR results, TPC2 protein was totally absent in TPC2 −/− MEFs in immunocytochemistry experiments, while it could be detected in wild-type (WT) MEFs ( Fig. 1b ). Western blot analysis of WT and TPC2 −/− liver samples confirmed absence of TPC2 protein in TPC2 −/− livers ( Supplementary Fig. 1b ). In lysosomes prepared from TPC2 −/− MEFs, currents elicited by postulated activators of TPC2, NAADP and PI(3,5)P 2 were strongly reduced ( Fig. 1c–e ). NAADP-dependent currents in WT lysosomes displayed a bell-shaped dose-response relationship ( Fig. 1d ) as reported previously [25] , [26] . 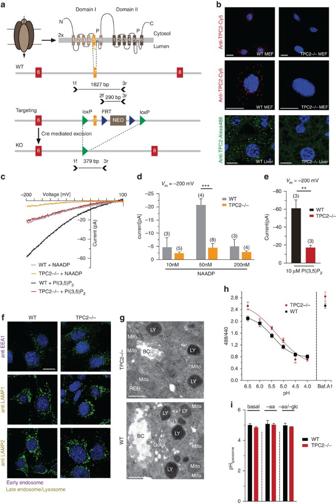Figure 1: Generation and characterization of TPC2 knockout mice. (a) Targeting strategy for the generation of TPC2−/−mice and validation. The targeted exon 7 of the mTPC2 gene encodes TMD5 and part of the pore-loop of domain I. Exons 6–8 are represented by boxes. The targeting vector contains twoloxPsites (green triangles), and a neo cassette flanked by two FLP recombination target (FRT) sites (blue triangles). (b) Representative immunofluroscence (IF) images of WT and TPC2−/−MEFs (stained with anti-TPC2 and Cy5) as well as WT and TPC2−/−liver cryosections (stained with anti-TPC2 and Alexa-488). Cell nuclei were visualized with Hoechst (MEFs) or 4',6-diamidino-2-phenylindole (DAPI) (liver). Scale bars, 20 μm. (c) Current–voltage relations of currents recorded from single-WT and -TPC2−/−lysosomes in the presence of 50 nM NAADP or 10 μM PI(3,5)P2. Lysosomes were isolated from vacuolin-treated WT and TPC2−/−MEFs before measurements. (d,e) Population data for current amplitudes at −200 mV obtained from experiments as shown ina; **P<0.01, ***P<0.001, two-way analysis of varicane (ANOVA) followed by Bonferroni’spost hoctest (d) or unpaired Student’st-test (e). (f) Expression and distribution of selected marker proteins for endosomes and lysosomes were unaffected in TPC2−/−compared with WT MEFs. Shown are representative confocal images of WT and TPC2−/−MEFs labelled with anti-EEA1, LAMP1 or LAMP2 and Alexa-488. Nuclei were visualized with DAPI. Scale bar, 20 μm. For additional markers, seeSupplementary Fig. 1. (g) Representative electron microscope images of WT and TPC2−/−liver sections. BC, bile canaliculus; LY, lysosome; Mito, mitochondrion; RER, rough endoplasmic reticulum. Scale bars, 500 nm. (h,i) Measurement of endolysosomal pH in WT and TPC2−/−cells. Late endocytic compartments of WT and TPC2−/−MEFs were labelled with dextran-Oregon Green 514. (h) Fluorescence intensity ratios were calculated for defined pH values as described in the Methods section. (i) Lysosomal pH values in WT and TPC2−/−MEFs were calculated using the calibration curves presented inhand determined under basal conditions, without amino acids (−aa, EBSS), and without both, aa and glucose (−aa, −glc). Baf. A1 was used as positive control; n.s., not significant, unpaired Student’st-test. Data points ind,e,handiare given as mean±s.e.m. Figure 1: Generation and characterization of TPC2 knockout mice. ( a ) Targeting strategy for the generation of TPC2 −/− mice and validation. The targeted exon 7 of the mTPC2 gene encodes TMD5 and part of the pore-loop of domain I. Exons 6–8 are represented by boxes. The targeting vector contains two loxP sites (green triangles), and a neo cassette flanked by two FLP recombination target (FRT) sites (blue triangles). ( b ) Representative immunofluroscence (IF) images of WT and TPC2 −/− MEFs (stained with anti-TPC2 and Cy5) as well as WT and TPC2 −/− liver cryosections (stained with anti-TPC2 and Alexa-488). Cell nuclei were visualized with Hoechst (MEFs) or 4',6-diamidino-2-phenylindole (DAPI) (liver). Scale bars, 20 μm. ( c ) Current–voltage relations of currents recorded from single-WT and -TPC2 −/− lysosomes in the presence of 50 nM NAADP or 10 μM PI(3,5)P 2 . Lysosomes were isolated from vacuolin-treated WT and TPC2 −/− MEFs before measurements. ( d , e ) Population data for current amplitudes at −200 mV obtained from experiments as shown in a ; ** P <0.01, *** P <0.001, two-way analysis of varicane (ANOVA) followed by Bonferroni’s post hoc test ( d ) or unpaired Student’s t -test ( e ). ( f ) Expression and distribution of selected marker proteins for endosomes and lysosomes were unaffected in TPC2 −/− compared with WT MEFs. Shown are representative confocal images of WT and TPC2 −/− MEFs labelled with anti-EEA1, LAMP1 or LAMP2 and Alexa-488. Nuclei were visualized with DAPI. Scale bar, 20 μm. For additional markers, see Supplementary Fig. 1 . ( g ) Representative electron microscope images of WT and TPC2 −/− liver sections. BC, bile canaliculus; LY, lysosome; Mito, mitochondrion; RER, rough endoplasmic reticulum. Scale bars, 500 nm. ( h , i ) Measurement of endolysosomal pH in WT and TPC2 −/− cells. Late endocytic compartments of WT and TPC2 −/− MEFs were labelled with dextran-Oregon Green 514. ( h ) Fluorescence intensity ratios were calculated for defined pH values as described in the Methods section. ( i ) Lysosomal pH values in WT and TPC2 −/− MEFs were calculated using the calibration curves presented in h and determined under basal conditions, without amino acids (−aa, EBSS), and without both, aa and glucose (−aa, −glc). Baf. A1 was used as positive control; n.s., not significant, unpaired Student’s t -test. Data points in d , e , h and i are given as mean±s.e.m. Full size image Expression and distribution of the early endosomal markers EEA1, Rab4 and Rab5, the late endosomal/lysosomal markers LAMP1, LAMP2, LIMP2 and CD63 or the recycling endosomal markers TfR, Rab4 and Rab11 were comparable in WT and TPC2 −/− cells ( Fig. 1f and Supplementary Fig. 1c–e ). Overexpression of the constitutively active Rab5 variant Rab5(Q79L) induced the formation of characteristic enlarged Rab5-positive vesicles both in WT and TPC2 −/− MEFs, indicating that early endosomal fusion is functioning normally ( Supplementary Fig. 1f ). Ultrastructural analyses of WT and TPC2 −/− liver samples using electron microscopy revealed no obvious alterations in the endolysosomal system ( Fig. 1g ). In particular, the number of endolysosomal vesicles did not show any deviations between the two genotypes. Notably, lysosomal deposits which have been reported in lysosomal storage diseases such as mucolipidosis type IV [27] , [28] could not be detected in TPC2 −/− mice. Finally, steady-state endolysosomal pH values were similar in TPC2 −/− and WT MEFs. This result was obtained in two different, independently generated WT and TPC2 −/− batches of MEFs: 5.08±0.1 for WT versus 4.93±0.06 for TPC2 −/− (batch-1) and 4.87±0.03 for WT versus 4.89±0.02 for TPC2 −/− (batch-2) ( Fig. 1h,i and Supplementary Fig. 1g–i ). Even under starvation conditions (EBSS buffer (−aa) or starvation buffer (−aa/−glc)), no significant differences in endolysosomal pH between WT and TPC2 −/− were observed (again two independently generated MEF cell lines (batch-1 and batch-2) were tested) ( Fig. 1i and Supplementary Table 1 ). In addition, the pH dependent, endolysosomal processing of cathepsin D and cathepsin L was examined. In the acidic environments of late endosomes and lysosomes, the mature forms of cathepsin D and cathepsin L are produced after proteolytic removal of the propeptide. We found that the generation of mature forms of cathepsin D and L was not impaired in TPC2 −/− MEFs compared with WT ( Supplementary Fig. 1j ). Specificity of the detected bands was controlled by analysing lysates from the respective cathepsin −/− MEFs in parallel. Next, we assessed the functional consequences of a loss of TPC2 for trafficking processes in the endolysosomal degradation pathway ( Fig. 2a ), the main subcellular localization of TPC2. This pathway can be tested by using labelled LDL which binds to its receptor and is internalized into the cell via endocytosis [10] . Subsequently, LDL dissociates from the receptor and is passed on to late endosomes and lysosomes, from where cholesterol is released into the cytosol ( Fig. 2a ). A trafficking or fusion defect within this pathway would lead to accumulation of LDL in vesicles proximal to the defect. We used LDL-BodipyFL to test this hypothesis and found that the number of LDL-positive vesicles per cell was significantly increased in TPC2 −/− compared with WT MEFs ( Fig. 2b–d ). This effect was observed at a broad range of LDL concentrations and after different pulse/chase times ( Fig. 2c,d ). LDLR expression in WT and TPC2 −/− MEFs was found to be similar as determined by quantitative western blot experiments (normalized to glyceraldehyde 3-phosphate dehydrogenase) ( Fig. 2e and Supplementary Fig. 2a ). As an independent test for the same pathway, we performed experiments using labelled EGF (epithelial growth factor; AlexaFluor488-EGF) [29] . These experiments revealed that EGF accumulation is increased in TPC2 −/− compared with WT MEFs ( Fig. 2f–h ). This finding was confirmed in independently generated MEFs (batch-2) ( Supplementary Fig. 2b,c ). In addition, in primary hepatocytes isolated from TPC2 −/− mice, the number of EGF-positive vesicles per cell was also significantly increased compared with WT hepatocytes, whereas EGFR expression in WT and TPC2 −/− livers was not significantly different ( Fig. 2i and Supplementary Fig. 2d,e ). To further assess whether the increased accumulation was caused by decreased degradation, the time course of EGF degradation after uptake was measured. MEFs were incubated with a saturating concentration of EGF (4 μg ml −1 ), followed by defined chase times before fixation ( Fig. 2j,k ). In TPC2 −/− MEFs, the fluorescence decreased significantly slower compared with WT MEFs. 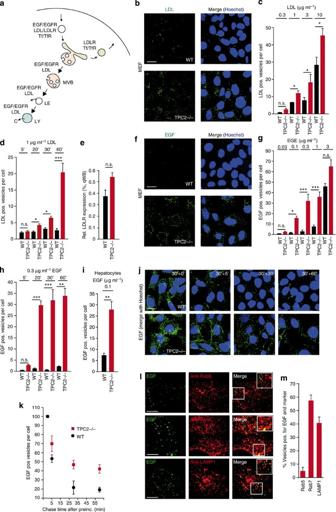Figure 2: TPC2 deletion leads to LDL and EGF/EGFR trafficking defects in the degradation pathway. (a) Cartoon illustrating endolysosomal degradation and recycling pathways. In the degradation pathway (endo/lysosomal axis) EGF/EGFR and LDL are degraded. In the recycling pathway LDLR and Tf/TfR are recycled. Cholesterol can exit the endolysosomal system from late endosomes or lysosomes. LE, late endosome; LY, lysosome; C, free cholesterol. (b) Representative confocal images of WT and TPC2−/−MEFs incubated with 3 μg ml−1LDL-BodipyFL. Cell nuclei were visualized with Hoechst. (c) Average numbers of LDL-positive vesicles per cell after an incubation time of 30 min at concentrations as indicated. (d) Average numbers of LDL-positive vesicles per cell after different incubation times at a concentration of 1 μg ml−1. (e) Quantitative western blot data showing average protein levels of LDLR in WT and TPC2−/−MEFs. (f) Representative confocal images of WT and TPC2−/−MEFs incubated with 0.3 μg ml−1AlexaFluor488-EGF. (g) Average numbers of EGF-positive vesicles per cell after an incubation time of 30 min at concentrations as indicated. (h) Average numbers of EGF-positive vesicles per cell after different incubation times at a concentration of 0.3 μg ml−1, followed by a 2-h chase period. (i) Average numbers of EGF-positive vesicles per cell from similar experiments with freshly prepared WT and TPC2−/−hepatocytes. (j) Representative confocal images of TPC2−/−and WT MEFs incubated with 4 μg AlexaFluor488-EGF for 30 min and chased for defined time intervals in EGF-free DMEM before fixation. (k) Time course of EGF degradation obtained from experiments as shown inj. (l) Representative confocal images of WT and TPC2−/−MEFs incubated with 1 μg ml−1AlexaFluor488-EGF for 30 min, fixed and stained with anti-LAMP1, anti-Rab5 and anti-Rab7 antibody, respectively, and Cy5 as secondery antibody. (m) Quantification of experiments as shown inl. All data points are given as mean±s.e.m. of at least three independent experiments, each. At least two independently generated WT and TPC2−/−MEF cell lines were analysed; n.s., not significant, ***P<0.001, **P<0.01, *P<0.05 (c,d,g,handk: two-way anlysis of variance (ANOVA) followed by Bonferroni’spost hoctest;eandi: unpaired Student’st-test). All scale bars, 20 μm. Figure 2: TPC2 deletion leads to LDL and EGF/EGFR trafficking defects in the degradation pathway. ( a ) Cartoon illustrating endolysosomal degradation and recycling pathways. In the degradation pathway (endo/lysosomal axis) EGF/EGFR and LDL are degraded. In the recycling pathway LDLR and Tf/TfR are recycled. Cholesterol can exit the endolysosomal system from late endosomes or lysosomes. LE, late endosome; LY, lysosome; C, free cholesterol. ( b ) Representative confocal images of WT and TPC2 −/− MEFs incubated with 3 μg ml −1 LDL-BodipyFL. Cell nuclei were visualized with Hoechst. ( c ) Average numbers of LDL-positive vesicles per cell after an incubation time of 30 min at concentrations as indicated. ( d ) Average numbers of LDL-positive vesicles per cell after different incubation times at a concentration of 1 μg ml −1 . ( e ) Quantitative western blot data showing average protein levels of LDLR in WT and TPC2 −/− MEFs. ( f ) Representative confocal images of WT and TPC2 −/− MEFs incubated with 0.3 μg ml −1 AlexaFluor488-EGF. ( g ) Average numbers of EGF-positive vesicles per cell after an incubation time of 30 min at concentrations as indicated. ( h ) Average numbers of EGF-positive vesicles per cell after different incubation times at a concentration of 0.3 μg ml −1 , followed by a 2-h chase period. ( i ) Average numbers of EGF-positive vesicles per cell from similar experiments with freshly prepared WT and TPC2 −/− hepatocytes. ( j ) Representative confocal images of TPC2 −/− and WT MEFs incubated with 4 μg AlexaFluor488-EGF for 30 min and chased for defined time intervals in EGF-free DMEM before fixation. ( k ) Time course of EGF degradation obtained from experiments as shown in j . ( l ) Representative confocal images of WT and TPC2 −/− MEFs incubated with 1 μg ml −1 AlexaFluor488-EGF for 30 min, fixed and stained with anti-LAMP1, anti-Rab5 and anti-Rab7 antibody, respectively, and Cy5 as secondery antibody. ( m ) Quantification of experiments as shown in l . All data points are given as mean±s.e.m. of at least three independent experiments, each. At least two independently generated WT and TPC2 −/− MEF cell lines were analysed; n.s., not significant, *** P <0.001, ** P <0.01, * P <0.05 ( c , d , g , h and k : two-way anlysis of variance (ANOVA) followed by Bonferroni’s post hoc test; e and i : unpaired Student’s t -test). All scale bars, 20 μm. Full size image To further determine the identity of the endolysosomal vesicles where EGF accumulates in TPC2 −/− cells, we co-labelled cells with markers for early endosomes (Rab5), late endosomes (Rab7), and late endosomes/lysosomes (LAMP1), and found that about 57% of the EGF-positive vesicles showed co-labelling with Rab7 and 41% with LAMP1, but only about 5% with Rab5, indicating that accumulation occurs rather in the late section of the endolysosomal system than in early endosomes ( Fig. 2l,m ). Taken together, these results suggested that EGF/EGFR and LDL-cholesterol transport and degradation are impaired in TPC2 −/− cells, and the endolysosomal transport machinery appeared to be saturated significantly faster in TPC2 −/− than in WT cells. Calcium and TPC2 channels are critical for trafficking Endolysosomal trafficking defects can be caused by multiple factors. They can result from defects in enzymatic degradation of macromolecules, which is the underlying cause of most lysosomal storage disorders. Impaired trafficking can also be caused by defects in the acidification of endolysosomal organelles, defective ionic homoeostasis or defects in endolysosomal fusion and fission processes. Defects in acidification of endolysosomal vesicles have been reported before to be the primary cause for the observed trafficking abnormalities for example, in mucolipidosis type IV, which is caused by mutations in the lysosomal cation channel TRPML1 (refs 27 , 30 , 31 ). However, endolysosmal pH appears normal in TPC2 −/− cells. Another attractive hypothesis for impaired endolysosomal trafficking is a defect in vesicle fusion or fission processes. It has been postulated before that Ca 2+ is required for vesicular fusion processes and thereby regulates trafficking of vesicular cargo proteins [30] , [32] , [33] . In accordance with this hypothesis, we found that in WT MEFs chelation of cytosolic Ca 2+ by 1,2-bis(2-aminophenoxy)ethane- N , N , N ′, N ′-tetraacetic acid tetrakis(acetoxymethyl ester) (BAPTA-AM) mimics the effect on EGF trafficking observed in TPC2 −/− MEFs ( Fig. 3a,b ). This effect was dose dependent ( Fig. 3a,b ). By contrast, in TPC2 −/− MEFs, EGF accumulation was not significantly changed by BAPTA-AM ( Fig. 3a,b ). Ethyleneglycol-bis( β -aminoethyl)- N , N , N ′, N ′-tetraacetoxymethyl ester (EGTA-AM), which has much slower binding kinetics than BAPTA-AM, had no significant effect on EGF accumulation ( Supplementary Fig. 2 ). 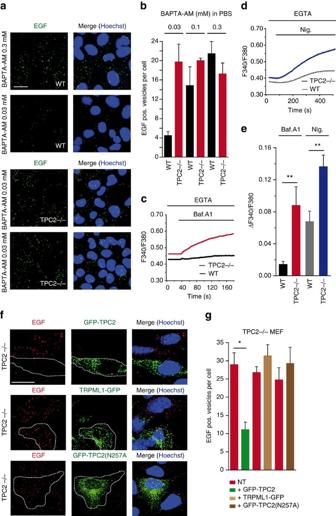Figure 3: Effects of BAPTA-AM or TPC2 overexpression on endolysosomal trafficking in WT and TPC2−/−MEFs. (a) Representative images of WT and TPC2−/−MEFs incubated with 0.1 μg ml−1AlexaFluor488-EGF (5 min), followed by an incubation with 0.1 μg ml−1AlexaFluor488-EGF in the presence of either 0.03 mM or 0.3 mM BAPTA-AM (25 min) in PBS. Cell nuclei were visualized with Hoechst. Scale bar, 20 μm. (b) Average numbers of AlexaFluor488-EGF-positive vesicles per cell after incubation with BAPTA-AM at different concentrations as described ina. (c,d) Effect of 2 μM bafilomycin A1 (Baf. A1;c) or 10 μM nigericin (Nig.;d) on cytosolic calcium levels in WT and TPC2−/−MEFs loaded with fura-2. Shown are representative calcium imging experiments (mean ofn=10 cells, each). Measurements were performed in the presence of 2 mM EGTA. (e) Summary of Baf. A1 and Nig. experiments; bars represent values 150 s (bafilomycin) or 450 s (nigericin) after compound application (n=at least five experiments with 5–10 cells, each). (f) TPC2 WT, the inactive TPC2 mutant TPC2(N257A), or TRPML1 WT were fused to green fluorescent protein (GFP), overexpressed in TPC2−/−MEFs and incubated with 1 μg ml−1AlexaFluor555-EGF (red). Shown are representative images after fixation of the respective MEF cell line as indicated. Cell nuclei were visualized with Hoechst. Scale bar, 20 μm. (g) Average numbers of EGF-positive vesicles per cell taken from experiments as shown ine. Non-transfected (NT) TPC2−/−cells in close proximity to cells transfected with the respective cDNAs served as positive controls for each experiment. All data points are given as mean±s.e.m. *P<0.05, **P<0.01, unpaired Student’st-test. Figure 3: Effects of BAPTA-AM or TPC2 overexpression on endolysosomal trafficking in WT and TPC2 −/− MEFs. ( a ) Representative images of WT and TPC2 −/− MEFs incubated with 0.1 μg ml −1 AlexaFluor488-EGF (5 min), followed by an incubation with 0.1 μg ml −1 AlexaFluor488-EGF in the presence of either 0.03 mM or 0.3 mM BAPTA-AM (25 min) in PBS. Cell nuclei were visualized with Hoechst. Scale bar, 20 μm. ( b ) Average numbers of AlexaFluor488-EGF-positive vesicles per cell after incubation with BAPTA-AM at different concentrations as described in a . ( c , d ) Effect of 2 μM bafilomycin A1 (Baf. A1; c ) or 10 μM nigericin (Nig. ; d ) on cytosolic calcium levels in WT and TPC2 −/− MEFs loaded with fura-2. Shown are representative calcium imging experiments (mean of n =10 cells, each). Measurements were performed in the presence of 2 mM EGTA. ( e ) Summary of Baf. A1 and Nig. experiments; bars represent values 150 s (bafilomycin) or 450 s (nigericin) after compound application ( n =at least five experiments with 5–10 cells, each). ( f ) TPC2 WT, the inactive TPC2 mutant TPC2(N257A), or TRPML1 WT were fused to green fluorescent protein (GFP), overexpressed in TPC2 −/− MEFs and incubated with 1 μg ml −1 AlexaFluor555-EGF (red). Shown are representative images after fixation of the respective MEF cell line as indicated. Cell nuclei were visualized with Hoechst. Scale bar, 20 μm. ( g ) Average numbers of EGF-positive vesicles per cell taken from experiments as shown in e . Non-transfected (NT) TPC2 −/− cells in close proximity to cells transfected with the respective cDNAs served as positive controls for each experiment. All data points are given as mean±s.e.m. * P <0.05, ** P <0.01, unpaired Student’s t -test. Full size image Bafilomycin A1 (Baf. A1)—a cell-permeant inhibitor of the vacuolar-type H + -ATPase, results in loss of the lysosomal/late endosomal proton gradient and eventually leads to the depletion of luminal calcium [34] . By using Baf. A1 (in the absence of extracellular calcium), we demonstrate that loss of TPC2 (TPC2 −/− MEF) causes a significant elevation in cytosolic calcium compared with WT, suggesting that loss of TPC2 may lead to an increased retention of calcium in the endolysosomal lumen ( Fig. 3c,e ). Similar results were obtained when the K + /H + exchanger nigericin was used instead of Baf. A1 (ref. 35 ) ( Fig. 3d,e ). Taken together, these results suggest that a significantly higher amount of calcium is retained in intracellular acidic compartments in TPC2 −/− compared with WT cells. To confirm that the Ca 2+ required for EGF trafficking depends on the presence of TPC2, we performed rescue experiments in TPC2 −/− MEFs and found that overexpression of WT TPC2 in TPC2 −/− MEFs leads to a rescue of the EGF-trafficking defects ( Fig. 3f,g ). The remaining EGF accumulation was not significantly different from the amount of EGF accumulating in WT MEFs at the respective EGF concentration ( Fig. 2g ). Notably, a non-conducting TPC2 mutant (TPC2-N257A) [21] was not sufficient to rescue trafficking defects, suggesting that ion flux through TPC2 is necessary for the rescue. Furthermore, the rescue is specific for TPC2 because TRPML1, another Ca 2+ permeable and PI(3,5)P 2 -activated cation channel in lysosomes [36] , did not rescue EGF-trafficking defects observed in TPC2 −/− MEFs ( Fig. 3f,g ). In vivo cholesterol accumulation in TPC2-deficient mice Given the pronounced impairments in LDL and EGF trafficking observed in TPC2 −/− MEF cell lines and hepatocytes, we hypothesized that defects might also be present in an in vivo model. Therefore, WT and TPC2 −/− mice were fed with a standard diet (SD) or a Western-type diet rich in cholesterol (CD) for 6 weeks, respectively [37] . Analysis of TPC2 −/− mice fed with SD indicated that these mice appeared identical to their WT littermates as determined by morphological and histological studies. The lack of a gross phenotype in TPC2 −/− mice on SD is not surprising, since SD contains relatively little cholesterol (≤0.02% w/w). On this diet, the cholesterol requirement of the animals is achieved primarily through de novo biosynthesis [38] . We next tested the effect of a diet rich in cholesterol (1.25% cholesterol; CD). The intake of cholesterol per day on this diet is approximately 20–30 times above the amount an average animal synthesizes to maintain homoeostasis when its dietary needs are not being met [38] . The average liver weight/body weight ratio of TPC2 −/− on CD was significantly increased compared with WT on CD ( Fig. 4a ), while this parameter was similar in WT and TPC2 −/− on SD. Importantly, there was no difference in total body weight between the two groups of mice, suggesting the absence of obesity in the TPC2 −/− mice. On macroscopic examination, more than 95% ( n =21) of TPC2 −/− livers (CD) displayed changes in colour ranging from slightly yellow to strongly yellow ( Fig. 4b,c ). Only about 5% of the livers looked normal. In contrast, 76% of WT livers (CD) looked normal while 24% displayed a light yellow colour ( n =21). Livers from WT and TPC2 −/− mice on SD did not display visible changes in colour ( n =13 and n =21, respectively). 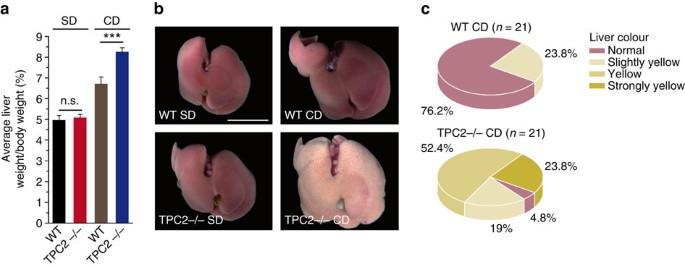Figure 4: Analysis of liver samples isolated from WT and TPC2−/−mice. (a) Bar diagram showing average liver weight/body weight ratios (in %) of WT and TPC2−/−mice treated for 6 weeks with SD or CD, respectively. **P<0.01, two-way analysis of variance (ANOVA) followed by Bonferroni’spost hoctest. (b) Shown are representative liver samples isolated from 10–12-week-old male WT and TPC2−/−mice, treated with either SD or CD for six consecutive weeks. Scale bar, 10 mm. (c) Pie charts showing the percentage of slightly to strongly yellow-stained liver samples isolated from WT and TPC2−/−mice treated with CD. Livers of SD-treated mice looked 100% normal. Figure 4: Analysis of liver samples isolated from WT and TPC2 −/− mice. ( a ) Bar diagram showing average liver weight/body weight ratios (in %) of WT and TPC2 −/− mice treated for 6 weeks with SD or CD, respectively. ** P <0.01, two-way analysis of variance (ANOVA) followed by Bonferroni’s post hoc test. ( b ) Shown are representative liver samples isolated from 10–12-week-old male WT and TPC2 −/− mice, treated with either SD or CD for six consecutive weeks. Scale bar, 10 mm. ( c ) Pie charts showing the percentage of slightly to strongly yellow-stained liver samples isolated from WT and TPC2 −/− mice treated with CD. Livers of SD-treated mice looked 100% normal. Full size image The prominent yellow colour of the livers from TPC2 −/− mice on CD is highly suggestive for hepatosteatosis (fatty liver). An analysis of the free and total hepatic cholesterol levels (free cholesterol and CEs) revealed that in SD-fed WT and TPC2 −/− mice, there was no difference in free and total liver cholesterol levels ( Fig. 5a–c ). After CD treatment, free and total cholesterol levels were elevated in both mouse lines. In TPC2 −/− mice, cholesterol levels were significantly higher than in WT mice ( Fig. 5a–c ). In particular, total cholesterol levels including CEs were dramatically increased in TPC2 −/− liver samples ( Fig. 5a–c ). In line with the biochemically observed hepatic overload of cholesterol and CEs in TPC2 −/− mice on CD, liver paraffin sections from TPC2 −/− mice on CD displayed strong accumulation of lipid droplets of different sizes predominantly in periportal hepatocytes ( Fig. 5d ). The histologic pattern is consistent with/resembles non-alcoholic fatty liver disease which is characterized by a microvesicular periportal hepatosteatosis. Signs of periportal and pericellular fibrosis were seen in liver sections from TPC2 −/− mice on CD ( Fig. 5e ). The strong accumulation of lipid droplets was further confirmed by electron microscopy of liver sections from TPC2 −/− mice on CD compared with WT on CD ( Fig. 5f ). Filipin [39] , [40] , [41] , [42] stainings further confirmed a strong accumulation of cholesterol in TPC2 −/− hepatocytes after CD treatment ( Fig. 6a ). A macroscopic analysis of gallbladders isolated from WT and TPC2 −/− mice on CD revealed the presence of large gallstones in TPC2 −/− gallbladders ( Supplementary Fig. 3a ). 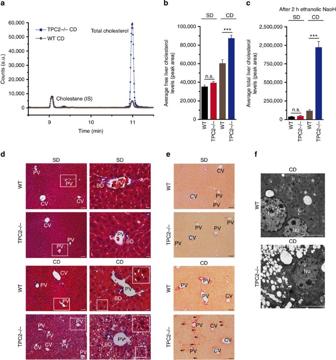Figure 5: Hepatic cholesterol overload, liver damage and hyperlipoproteinaemia in TPC2−/−mice. (a) Representative gas chromatogram (m/z217+368) of total cholesterol and internal standard (IS) after alkaline hydrolysis in liver tissue prepared from male WT and TPC2−/−mice on CD. (b) Average hepatic levels of unesterified free cholesterol in male WT and TPC2−/−mice on SD or CD as indicated (GC split ratio 3). (c) Average total liver cholesterol levels, determined after alkaline ester hydrolysis (GC split ratio 15). (d) Representative images of liver paraffin sections of male WT and TPC2−/−mice on SD or CD diet, respectively, stained with haematoxylin–eosin (HE). BD, bile duct; PV, portal vein; CV, central vein. Scale bars, 100 μm (SD left, CD left) and 20 μm (SD right, CD right). White arrows point to some lipid droplets visible in CD WT sections. (e) Representative images of liver paraffin sections stained with Sirius Red. PV, portal vein; CV, central vein. Scale bars, 100 μm. Black arrows point to areas of pericellular fibrosis in CD-treated TPC2−/−livers. (f) Representative electron microscope images of WT and TPC2−/−liver sections after CD treatment. Nu, nucleus; scale bars, 5 μm. Data points inbandcare given as mean±s.e.m. (bandc: two-way analysis of variance (ANOVA) followed by Bonferroni’spost hoctest; n.s., not significant, ***P<0.001. Figure 5: Hepatic cholesterol overload, liver damage and hyperlipoproteinaemia in TPC2 −/− mice. ( a ) Representative gas chromatogram ( m/z 217+368) of total cholesterol and internal standard (IS) after alkaline hydrolysis in liver tissue prepared from male WT and TPC2 −/− mice on CD. ( b ) Average hepatic levels of unesterified free cholesterol in male WT and TPC2 −/− mice on SD or CD as indicated (GC split ratio 3). ( c ) Average total liver cholesterol levels, determined after alkaline ester hydrolysis (GC split ratio 15). ( d ) Representative images of liver paraffin sections of male WT and TPC2 −/− mice on SD or CD diet, respectively, stained with haematoxylin–eosin (HE). BD, bile duct; PV, portal vein; CV, central vein. Scale bars, 100 μm (SD left, CD left) and 20 μm (SD right, CD right). White arrows point to some lipid droplets visible in CD WT sections. ( e ) Representative images of liver paraffin sections stained with Sirius Red. PV, portal vein; CV, central vein. Scale bars, 100 μm. Black arrows point to areas of pericellular fibrosis in CD-treated TPC2 −/− livers. ( f ) Representative electron microscope images of WT and TPC2 −/− liver sections after CD treatment. Nu, nucleus; scale bars, 5 μm. Data points in b and c are given as mean±s.e.m. ( b and c : two-way analysis of variance (ANOVA) followed by Bonferroni’s post hoc test; n.s., not significant, *** P <0.001. 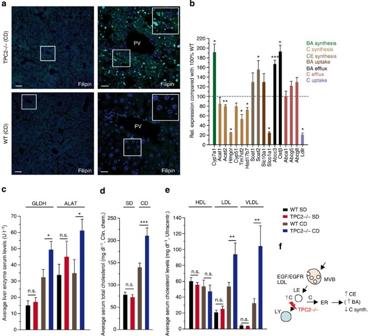Figure 6: Cholesterol accumulation in liver tissue isolated from TPC2−/−and WT mice and gene expression profile. (a) Representative images of liver cryosections of WT and TPC2−/−mice on CD diet, stained with filipin (0.05 mg ml−1in PBS for 2 h) to visualize free cholesterol. Scale bars, 100 μm (left) and 20 μm (right). (b) Relative expression (WT compared with TPC2−/−on CD) of hepatic transcripts coding for proteins involved in: bile acid (BA) synthesis (Cholesterol-7-alpha-hydroxylase, Cyp7a1), cholesterol synthesis (Acat1 (acetyl-CoA acetyltransferase 1, mitochondrial), Acat2 (acetyl-CoA acetyltransferase 2, cytosolic), Hmgcr (HMG-CoA reductase), Cyp51 (Lanosterol 14α-demethylase), Tm7sf2 (delta(14)-sterol reductase), cholesterol ester (CE) synthesis (Soat1 and Soat2 (sterol O-acyltransferase 1 and 2)), BA efflux (Abcc3 (canalicular multispecific organic anion transporter 2), Ostβ (organic solute transporter beta)), BA uptake (Slc10a1 (Na+-taurocholate cotransporting polypeptide, Ntcp), Slco1a1 (organic anion-transporting polypeptide, Oatp), sterol/cholesterol efflux transporters (Abca1, Abcg5, Abcg8) and cholesterol uptake (Ldlr). *P<0.05, **P<0.01, ***P<0.001, unpaired Student’st-test. Expression of Hmgcr and Ldlr was determined by quantitative RT–PCR and normalized to beta actin. (c) Average liver enzyme levels (GLDH (glutamate dehydrogenase) and ALAT (alanine transaminase) in male WT and TPC2−/−mice on SD or CD as indicated. (d) Average serum total cholesterol levels in male WT and TPC2−/−mice on SD or CD. (e) Average HDL-, LDL- and VLDL-cholesterol levels in serum of male WT and TPC2−/−mice on SD or CD diet. **P<0.01, ***P<0.001, two-way analysis of variance (ANOVA) followed by Bonferroni’spost hoctest; n.s., not significant. (f) Cartoon illustrating hypothetical model of cholesterol accumulation. Cholesterol accumulates in LEs in TPC2−/−cells due to a delay or impairment of LE/LY fusion/trafficking processes (symbolized by the red flash); C, free cholesterol; CE, cholesterol ester; BA, bile acid. All data points are given as mean±s.e.m. Full size image Figure 6: Cholesterol accumulation in liver tissue isolated from TPC2 −/− and WT mice and gene expression profile. ( a ) Representative images of liver cryosections of WT and TPC2 −/− mice on CD diet, stained with filipin (0.05 mg ml −1 in PBS for 2 h) to visualize free cholesterol. Scale bars, 100 μm (left) and 20 μm (right). ( b ) Relative expression (WT compared with TPC2 −/− on CD) of hepatic transcripts coding for proteins involved in: bile acid (BA) synthesis (Cholesterol-7-alpha-hydroxylase, Cyp7a1), cholesterol synthesis (Acat1 (acetyl-CoA acetyltransferase 1, mitochondrial), Acat2 (acetyl-CoA acetyltransferase 2, cytosolic), Hmgcr (HMG-CoA reductase), Cyp51 (Lanosterol 14α-demethylase), Tm7sf2 (delta(14)-sterol reductase), cholesterol ester (CE) synthesis (Soat1 and Soat2 (sterol O-acyltransferase 1 and 2)), BA efflux (Abcc3 (canalicular multispecific organic anion transporter 2), Ostβ (organic solute transporter beta)), BA uptake (Slc10a1 (Na + -taurocholate cotransporting polypeptide, Ntcp), Slco1a1 (organic anion-transporting polypeptide, Oatp), sterol/cholesterol efflux transporters (Abca1, Abcg5, Abcg8) and cholesterol uptake (Ldlr). * P <0.05, ** P <0.01, *** P <0.001, unpaired Student’s t -test. Expression of Hmgcr and Ldlr was determined by quantitative RT–PCR and normalized to beta actin. ( c ) Average liver enzyme levels (GLDH (glutamate dehydrogenase) and ALAT (alanine transaminase) in male WT and TPC2 −/− mice on SD or CD as indicated. ( d ) Average serum total cholesterol levels in male WT and TPC2 −/− mice on SD or CD. ( e ) Average HDL-, LDL- and VLDL-cholesterol levels in serum of male WT and TPC2 −/− mice on SD or CD diet. ** P <0.01, *** P <0.001, two-way analysis of variance (ANOVA) followed by Bonferroni’s post hoc test; n.s., not significant. ( f ) Cartoon illustrating hypothetical model of cholesterol accumulation. Cholesterol accumulates in LEs in TPC2 −/− cells due to a delay or impairment of LE/LY fusion/trafficking processes (symbolized by the red flash); C, free cholesterol; CE, cholesterol ester; BA, bile acid. All data points are given as mean±s.e.m. Full size image To test whether the severe cholesterol overload of TPC2 −/− livers causes compensatory hepatic changes, a pathway analysis of differentially regulated genes was performed in TPC2 −/− and WT mice on SD and CD diet. This analysis revealed significant enrichment of genes involved in lipid metabolism and molecular transport ( Supplementary Table 2 ). In line with an increased hepatic pool of free cholesterol, transcriptional upregulation of hepatic enzymes involved in BA and CE synthesis as well as BA efflux was observed in TPC2 −/− compared with WT mice on CD, while enzymes involved in hepatic cholesterol synthesis were downregulated ( Fig. 6b ) [43] , [44] , [45] . LDLR expression levels were comparable in livers from WT and TPC2 −/− mice on SD (data not shown), while a significant downregulation was observed in livers from TPC2 −/− mice on CD compared with WT on CD ( Fig. 6b ). Expression of the ABC transporters ABCA1, ABCG5 (sterolin-1) and ABCG8 (sterolin-2) was not significantly upregulated ( Fig. 6b ). An analysis of faecal BA content and composition revealed an increase in BA excretion in CD compared with SD-fed animals, which was, however, independent of the genotype ( Supplementary Fig. 3b ). In liver, only one type of BA was consistently detectable: cholic acid. While desoxycholic acid was not detectable in liver samples of SD-fed animals, it was detectable in 40% of the investigated CD-fed TPC2 −/− animals ( Supplementary Fig. 3c ). We further assessed functional hepatic consequences of the measured cholesterol accumulation by determining liver-specific enzyme levels in the peripheral blood. While no differences in enzyme levels indicating liver damage such as glutamate dehydrogenase or alanine transaminase were found in mice on SD, significantly increased glutamate dehydrogenase and alanine transaminase values ( Fig. 6c and Table 1 ) were detected in TPC2 −/− mice compared with WT on CD. Taken together, these findings indicate that in addition to hepatic cholesterol overload, liver damage was present in TPC2 −/− mice after CD treatment. Table 1 Summary of serum parameters. Full size table Since the liver is the key organ in regulating lipoprotein metabolism, we next determined systemic changes in lipoproteins. In WT and TPC2 −/− mice fed with SD, we found no differences in total cholesterol as well as HDL- (high-density lipoprotein), LDL- or VLDL-cholesterol (very low-density lipoprotein cholesterol) plasma levels ( Fig. 6d,e ). However, in mice on CD, total blood cholesterol levels as well as LDL- and VLDL-cholesterol levels were strongly elevated. Notably, LDL- and VLDL-cholesterol levels were significantly more increased in TPC2 −/− than in WT mice. Serum HDL-cholesterol levels as well as protein, triglyceride and glucose levels were similar within both groups ( Table 1 ). Finally, faecal total cholesterol levels were increased in CD compared with SD-fed animals. However, here no significant differences were detectable between the genotypes ( Supplementary Fig. 3d ). Here, we show that TPC2 −/− mice are more susceptible to cholesterol and CE accumulation in the liver than WT mice. This accumulation is not caused by extrahepatic factors, because similar accumulation is seen in single-cell experiments. The macroscopic and histological presentation of TPC2 −/− livers, the increased cholesterol accumulation and increase in hepatic transaminases indicate fatty liver and liver damage, and are consistent with the clinical picture of NAFLD and NASH. The clinical phenotype can be explained by specific defects in vesicle trafficking along the endolysosomal degradation pathway in the TPC2 −/− mouse. In the absence of TPC2, receptors and cargoes such as LDL or EGF/EGFR, which are transported along the degradation pathway, accumulate rapidly in intracellular vesicles of TPC2 −/− but not WT cells. This finding suggests that TPC2 channels are critically involved in the regulation of endolysosomal trafficking along this pathway. Since TPC2 channels are specifically expressed on late endosomes and lysosomes, it is likely that TPC2 regulates or enhances the final transport or fusion step between these two organelles. Consistent with this hypothesis, deletion of TPC2 leads to a partial block in transport and accumulation of LDL-cholesterol and LDL CEs proximal to the fusion defect in the prelysosomal vesicle pool, in particular late endosomes ( Fig. 6f ). LDL-derived CEs are normally hydrolysed to free cholesterol by lysosomal and late endosomal acid lipase and subsequently exported from the endolysosomal system. Due to prelysosomal accumulation, more cholesterol may exit via late endosomes in TPC2 −/− mice and thus increase the free cholesterol pool in the cytosol. It is well known that an increased free cholesterol pool at the endoplasmic reticulum (ER) induces CE formation and deposition in lipid droplets as well as downregulation of endogenous cholesterol synthesis ( Fig. 6f ) [43] , [44] . In line with this theory, we found that CEs are increased in TPC2 −/− mice. CEs are generated from free cholesterol by Soat1 and Soat2 (sterol O-acyltransferase 1 and 2). These enzymes are upregulated in livers of TPC2 −/− mice. ER enzymes involved in endogenous cholesterol synthesis are downregulated. Finally, serum VLDL levels are elevated in TPC2 −/− mice on CD ( Fig. 6e ). While this elevation could be caused by an increase in hepatic VLDL production, the possibility of a reduced VLDL clearance cannot completely be ruled out. Together, these results indicate that in TPC2 −/− hepatocytes, secondary ER-dependent processes are induced. This could either be caused by a globally increased free cholesterol pool or alternatively by misrouting of free cholesterol to the ER. Such a misrouting effect could be caused by a decreased flux of cholesterol from late endosomes to lysosomes with an upregulation of alternative trafficking pathways from late endosomes to the ER. In support of this notion, there is increasing evidence of contact sites between late endosomes and the ER [46] , [47] , [48] , as well as evidence for direct vesicular and non-vesicular transport of cholesterol to the ER from late endosomes [49] , [50] . How could a proposed role of TPC2 for vesicular trafficking and fusion be explained mechanistically? We demonstrate that in MEFs, TPC2 is critically involved in the generation of a current specifically activated by the known TPC2 activators NAADP and PI(3,5)P 2 . It has been shown that PI(3,5)P 2 concentrations increase from early to late endosomes [9] , [11] , [15] . Thus, in the absence or in the presence of very low levels of PI(3,5)P 2 , TPC2 may conduct only very small currents and progressively start to open on maturation toward late endosomes as PI(3,5)P 2 gradually rises. Opening of TPC2 channels in late endosomes could initiate the final fusion between late endosomes and lysosomes. Here, we demonstrate that vesicle trafficking in the endo/lysosomal degradation pathway requires Ca 2+ and ion flux through TPC2. The most likely interpretation is that Ca 2+ flows directly through TPC2 channels. TPC2 has been shown previously to conduct Ca 2+ (refs 18 , 21 , 22 , 24 ) and we confirm here that endogenous TPC2 channels are permeable to calcium ( Supplementary Fig. 4 ). Opening of TPC2 channels may lead to Ca 2+ efflux from vesicles directly into microdomains surrounding Ca 2+ -dependent proteins of the fusion machinery and thereby induce fusion. Anchoring of TPC2 within the cellular fusion machinery is supported by interactions with specific SNARE proteins such as STX7 and additional protein components of SNARE complexes which were identified by proteomics-based interaction screens, and confirmed by fluorescence resonance energy transfer analyses and co-immunoprecipitation experiments ( Supplementary Fig. 5a–g and Supplementary Table 3 ) [51] , [52] , [53] . Alternatively, ionic flux through TPC2 channels could also be part of an indirect mechanism which provides Ca 2+ . In this scenario, cations other than Ca 2+ flowing through TPC2 would act on a downstream channel, which in turn provides Ca 2+ . Na + and K + have also been shown to permeate through TPC2 channels [17] , [20] . Given the proposed close structural assembly of TPCs and the fusion machinery ( Supplementary Fig. 5g ), depolarization by Na + efflux through TPC2 may also electrostatically facilitate fusion between two vesicular membranes as suggested by the model of Wang et al. [17] Similar events may be relevant for TPC1 within the proximal endosomal pathway. Defects in the endolysosomal trafficking and cellular processing of LDL-cholesterol have been implicated in human diseases such as Niemann Pick disease and Wolman’s disease (CE storage disease) where CEs accumulate in late endosomes and lysosomes due to a severely diminished activity of cholesterol export proteins NPC1 and NPC2 or lysosomal acid lipase [54] . Here, we demonstrate that loss of TPC2 results in a defect which is more distally located in the endolysosomal LDL-cholesterol trafficking pathway. Loss of TPC2 increases the risk of developing NAFLD and NASH. These diseases themselves are independent of traditional cardiovascular risk factors and the metabolic syndrome associated with increased risk for cardiovascular disease. Furthermore, in obese individuals these diseases are markers of insulin resistance and diabetes. Notably, TPC2 −/− mice are highly susceptible to NAFLD and NASH, while obesity and impaired glucose tolerance are not observed. This finding suggests that TPC2 −/− mice have a reduced metabolic reserve in hepatic cholesterol handling, which leads to NAFLD even in the absence of obesity and impaired glucose tolerance. The increased susceptibility of TPC2 −/− mice to NAFLD is clinically highly relevant because this disease affects up to one-third of the population worldwide and may cause adverse cardiovascular outcome and increased cardiovascular mortality. Generation of TPC2 −/− knockout mice TPC2 −/− mice were generated by deleting exon 7 and introducing an early stop codon. We generated a targeting vector that, after homologous recombination, resulted in a modified TPC2 allele carrying two loxP sites flanking exon 7. A neo R cassette, which was used for G418/geneticin selection, was removed with Flp recombinase before the ES cells were injected into host blastocysts to generate chimeric mice. After germline transmission and continued breeding, PCR with genomic DNA from progeny of WT, heterozygous and homozygous animals showed proper recombination and inheritance of the TPC2 lox allele. Subsequently, exon 7 was deleted by pairing TPC2 lox mice with mice expressing Cre-recombinase under a cytomegalovirus promoter. Exon 7 encodes TMD5 and part of the pore-loop in domain I of TPC2. Animals were used under approved animal protocols and University of Munich (LMU) Institutional Animal Care Guidelines. Whole-lysosome planar patch-clamp experiments For whole-lysosome planar patch-clamp recordings, isolated intact lysosomes from HEK293 cells or MEFs were prepared by differential centrifugation as described previously [21] , [22] , [55] . HEK293 cells stably expressing murine TPC2 or the TPC2 mutant TPC2(N257A), both N-terminally fused to green fluorescent protein and subcloned into pcDNA5FRT vector with hygromycin resistance (Invitrogen) were used. To investigate STX7 effects on TPC2, a double stable HEK293 cell line was generated coexpressing murine STX7, N-terminally fused to mCherry (in pcDNA3 vector with geneticin (G418) resistance) and TPC2 as described above. The planar patch-clamp technology combined with a fast internal perfusion system (Port-a-Patch, Nanion Technologies) was applied as described previously [21] , [22] , [55] . Currents were recorded using an EPC-10 patch-clamp amplifier and PatchMaster acquisition software (HEKA). Data were digitized at 40 kHz and filtered at 2.8 kHz. Mean endolysosomal capacitance was 1.01±0.04 pF ( n =47). For all experiments, salt-agar bridges were used to connect the reference Ag-AgCl wire to the bath solution to minimize voltage offsets. Unless otherwise stated, cytoplasmic solution contained 60 mM KF, 70 mM K-MSA (methanesulfonate), 0.2 mM Ca-MSA, 4 mM Na-MSA, 10 mM HEPES (pH adjusted with KOH to 7.2). Luminal solution was 60 mM Ca-MSA, 85 mM Na-MSA, 1 mM MgCl 2 , 10 mM HEPES (pH adjusted with NaOH to 4.6 (refs 17 , 20 )). Mannitol was used to adjust osmolarity. For the application of PI(3,5)P 2 (A.G. Scientific) or NAADP (Tocris Bioscience), cytoplasmic solution was completely exchanged by PI(3,5)P 2 - or NAADP-containing solution. Endolysosomal trafficking experiments For trafficking experiments, AlexaFluor488-EGF, AlexaFluor555-EGF or LDL-BodipyFL (Life Technologies) were used. MEFs from WT and TPC2 −/− mice were seeded on glass coverslips in 24-well plates and grown in Dulbeccos modified eagles medium (DMEM) with 10% fetal bovine serum at 37 °C and 5% CO 2 for 48 h. Cells were treated with varying concentrations of labelled LDL or EGF and incubated for different time intervals at 37 °C and 5% CO 2 . Cells were subsequently washed in DMEM containing no fetal bovine serum and fixed with ice-cold methanol for 5 min at −20 °C or chased before fixation for defined time intervals at 37 °C and 5% CO 2 in DMEM containing no fetal bovine serum, as indicated in the respective figure legends. Hoechst nuclear staining (Hoechst 33342) was performed in PBS buffer (5 μg ml −1 ). Cells were incubated at room temperature for another 30 min, washed twice with PBS and embedded in Cell Lab Fluoromount-G Slide Mounting Medium (Beckman Coulter). In the degradation format, cells were incubated as described above with a saturating concentration of AlexaFluor488-EGF (4 μg ml −1 ) for 30 min, washed and incubated for different chase times as indicated. For data quantification, ImageJ software was used. In each experiment, numbers were calculated based on the total number of vesicles (dots) per image divided by the number of cells (nuclei) per image. The term ‘cell’ is used instead of ‘confocal cell section’. Endolysosomal pH measurements Endolysosomal pH measurements were performed by ratiometric fluorescence imaging as described previously [56] . MEFs were seeded on imaging dishes (145 μm glass bottom, PAA Laboratories, Germany) and grown overnight in DMEM supplemented with 1 g l −1 bovine serum albumin in the presence of 500 μg ml −1 of the pH-sensitive fluorophore Oregon Green 514 conjugated to dextran (70,000 MW, Life Technologies). In order to allow clearance of early endocytic compartments and ensure specific localization of the dye in the late endocytic pathway, cells were chased in DMEM at 37 °C for 1 h in the presence of bovine serum albumin followed by 1-h incubation in serum-free medium before imaging for basal pH determination. To assess lysosomal pH under starvation conditions, the chase procedure was replaced by either 2-h incubation without amino acids (EBSS) or 2-h incubation without both, amino acids and glucose (110 mM NaCl, 45 mM NaHCO 3 , 5 mM KCl, 2 mM CaCl 2 , 1 mM MgCl 2 , pH 7.4) [20] . As a control for increased lysosomal pH, 200 nM Baf. A1 (Sigma Aldrich) were applied during the 1-h incubation in serum-free medium under basal conditions. Ratiometric imaging was performed using an Olympus FV1000 confocal laser scanning microscope. Cells were excited alternately by light transmitted from a 440-nm laser diode or a multiline argon laser at 488 nm (Showa electronics model GLS3135). In both cases, images were acquired at an emission wavelength of 535±20 nm using a charge-coupled device-camera. At the end of every experiment, an in situ calibration was performed for each genotype by incubating the cells with isotonic K + buffer solutions (145 mM KCl, 10 mM glucose, 1 mM MgCl 2 and 20 mM of either HEPES, MES or acetate, pH ranging from 4.0 to 7.0), containing 10 μg ml −1 of the ionophorenigericin. The resulting fluorescence intensity ratios (488/440) were fitted to the Boltzmann equation to interpolate pH values from the experimental ratio data. Calcium imaging experiments Calcium imaging experiments were performed using fura-2 as described previously [57] . Briefly, WT and TPC2 −/− MEFs cells were plated onto glass coverslips, and after 24 h, cells were loaded for 1 h with the fluorescent indicator fura-2-AM (4 μM; Invitrogen) in a standard bath solution containing (in mM) 138 NaCl, 6 KCl, 2 MgCl 2 , 2 CaCl 2 , 10 HEPES and 5.5 D-glucose (adjusted to pH 7.4 with NaOH). Cells were washed in 2 mM EGTA for 30 min before measurement. Calcium imaging was performed using a monochromator-based imaging system (Polychrome IV monochromator, TILL Photonics). Compounds were applied in the presence of 2 mM EGTA. Immunocyto- and immunohistochemistry, electron microscopy Immunocytochemistry was performed as described previously [58] . Histology, immunohistochemistry and electron microscopy experiments were performed according to standard protocols. For further details, please refer to Supplementary methods . Serum cholesterol levels and expression profiling in liver Male TPC2 −/− and WT mice were fed with standard chow diet (SD) or a high-cholesterol containing Western-type diet (1.25% cholesterol, 15% fat, 0.5% Na-cholate; ssniff GmbH, Soest, Germany) for 6 weeks. Throughout the text, we refer to this diet by calling it cholesterol diet or CD. On the day of euthanasia, food was removed from the cage and approximately 8 h later, mice were killed as described [59] and blood was drawn by left-ventricular puncture in EDTA-containing syringes. Cell counting was performed after 1:4 dilution with PBS in an automated hematology analyzer (Sysmex). Lipoproteins were isolated by sequential ultracentrifugation from 60 μl of plasma at d <1.006 g ml −1 (VLDL) 1.006≤ d ≤1.063 g ml −1 (intermediate- and low-density lipoprotein (IDL and LDL, respectively)) and d >1.063 g ml −1 (high-density lipoprotein (HDL)) in a TL100 ultracentrifuge (Beckman). Cholesterol was determined enzymatically by using a colorimetric method (Roche). RNA from liver samples of TPC2 −/− and WT mice fed with SD (WT n =4; TPC2 −/− n =4) or CD (WT n =4; TPC2 −/− n =4) was isolated as described previously [60] . RNA was labelled and hybridized to Illumina Mouse Ref-8 v2.0 Expression Bead Chips and arrays were scanned with an Illumina iScan microarray scanner. Bead level data pre-processing was done in Illumina Genome Studio followed by quantile normalization and background reduction according to standard procedures in the software. Of the >25,600 annotated RefSeq transcripts that were covered by the arrays, a total of 4,598 transcripts were upregulated or downregulated in TPC2 −/− mice with fold changes >20% compared with WT control. Of these, 2,159 transcripts were differentially regulated in livers of mice on SD and 3,288 partially overlapping transcripts were differentially regulated in livers of mice on CD. Using the Ingenuity Pathways Analysis software ( www.ingenuity.com ), most significantly enriched biological functions in WT and TPC2 −/− mice were identified and levels of significance were determined using Fisher’s exact tests implemented in the software [61] . Alternatively, expression of Ldlr (5′-primer 5′-TGGGTCATCGCCCTGCT-3′, 3′-primer 5′-TTCCTGCTGCATGAGTCTTCT-3′, probe 5′FAM-5′-CTGGCTGCTGCCGGAGTTGCA-3′TAMRA), Egfr (5′-primer 5′-CCTATGCCACGCCAACTGTAC-3′, 3′-primer 5′-GATGGCCACACTTCACATCCT-3′, probe 5′FAM-5′-TATGGATGTGCTGGGCCAGGTCTTC-3′TAMRA) was assessed in liver samples by quantitative RT–PCR and normalized to glyceraldehyde 3-phosphate dehydrogenase (5′-primer 5′-TGTCCGTCGTGGATCTGACG-3′, 3′-primer 5′-CCAAGATGCCCTTCAGTGGG-3′, probe 5′FAM-5′-CGCCTGGAGAAACCTGCCAAGTATGATGAC-3′TAMRA). Determination of hepatic cholesterol by gas chromatography mass spectrometry Gas chromatography mass spectrometry analysis was performed on a Varian 3800 gas chromatograph coupled with a Varian Saturn 2200 ion trap. The stationary phase was an Agilent VF-5 ms capillary column with 30 m × 0.25 mm inner diameter and 0.25 μm film thickness. The mobile phase was helium at a constant flow rate of 1.4 ml min −1 . The inlet temperature was 250 °C, injection volume 1 μl (split ratio 3 for free liver cholesterol and 15 for total liver cholesterol after alkaline ester hydrolysis). The GC oven started at 70 °C, ramped up to 270 °C (heating rate 50 °C min −1 ), followed by a gradient of 5 °C min −1 up to 310 °C. Transfer line temperature was 270 °C and the ion-trap temperature was 200 °C. MS scanned from 8.5 to 12.0 min at a mass range of 100–550 m/z (electron ionization, 70 eV). The peak areas of characteristic ions forcholesterol tetramethylsilane ether (368 m/z ) and for cholestane (217 m/z ) were used for data analysis. The mean value of each double-injected sample ( n =5) was used for statistical analysis. For details of sample preparation, please refer to Supplementary methods . Statistical analysis Details of statistical analyses and n values are provided in the methods subsections or the figure legends. Statistical analyses were carried out using Origin 7.5 and GraphPad Prism 5. All error bars are depicted as mean±s.e.m. Statistical significance was determined via Student’s t -test, one-way analysis of variance followed by Tukey’s post test, or two-way analysis of variance followed by Bonferroni’s post hoc test, unless stated otherwise. Significance is denoted on figures as outlined in the legends. Statistics were derived from at least three independent experiments. How to cite this article: Grimm, C. et al. High susceptibility to fatty liver disease in two-pore channel 2-deficient mice. Nat. Commun. 5:4699 doi: 10.1038/ncomms5699 (2014).